Correspondence: Reply to ‘Enhancing a phase measurement by sequentially probing a solid-state system’ 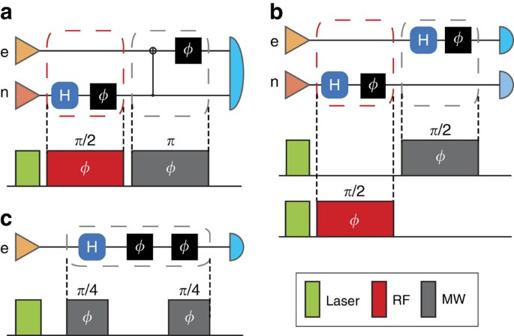Figure 1: The quantum circuits and pulse sequences in our experiment. (a) The entanglement-enhanced strategy applied in our experiment. (b) The classical strategy applied in our experiment. (c) The possible sequential strategy in our set-up. The triangles on the left represent state preparation and the symbols on the right represent measurements. The grey boxes represent a unitary operation involving multiple probes3. How to cite this article: Liu, G-Q. et al . Correspondence: Reply to ‘Enhancing a phase measurement by sequentially probing a solid-state system’. Nat. Commun. 7:11521 doi: 10.1038/ncomms11521 (2016).